Tuning organic magnetoresistance in polymer-fullerene blends by controlling spin reaction pathways Harnessing the spin degree of freedom in semiconductors is generally a challenging, yet rewarding task. In recent years, the large effect of a small magnetic field on the current in organic semiconductors has puzzled the young field of organic spintronics. Although the microscopic interaction mechanisms between spin-carrying particles in organic materials are well understood nowadays, there is no consensus as to which pairs of spin-carrying particles are actually influencing the current in such a drastic manner. Here we demonstrate that the spin-based particle reactions can be tuned in a blend of organic materials, and microscopic mechanisms are identified using magnetoresistance lineshapes and voltage dependencies as fingerprints. We find that different mechanisms can dominate, depending on the exact materials choice, morphology and operating conditions. Our improved understanding will contribute to the future control of magnetic field effects in organic semiconductors. The field of organic spintronics deals with spin physics and magnetic field effects (MFEs) in organic materials [1] , [2] . Besides spin injection into organic semiconductors [3] , [4] , a lot of attention was drawn to non-spin-polarized organic semiconductor device. Despite the absence of magnetic elements, they show a large room-temperature magnetoresistance effect at relatively small magnetic fields of only a few millitesla, an effect sometimes referred to as organic magnetoresistance (OMAR) [5] , [6] , [7] , [8] , [9] , [10] , [11] , [12] , [13] , [14] , [15] , [16] , [17] , [18] , [19] , [20] , [21] , [22] . Cheap plastic sensor technology has been suggested as an example of its application potential [23] . However, because this MFE was discovered a decade ago, the desire to unravel the exciting new physics behind the intrinsically magnetic field-dependent charge-transport properties of organic semiconductors has been the major motivation for intensive experimental [5] , [6] , [7] , [8] , [9] , [10] , [11] , [12] , [13] , [14] and theoretical [15] , [16] , [17] , [18] , [19] , [20] , [21] , [22] research. Several mechanisms have been suggested to explain OMAR. All these mechanisms rely on spin-selective reactions between pairs of particles, where a magnetic field suppresses the spin mixing of the particle pairs before the reaction, thereby changing the spin fraction and the outcome. Partly based on recent studies—where the MFEs from standard and deuterated polymers were compared—there is a growing consensus about the importance of hyperfine fields (hfs) for spin mixing [12] . The principal question in the field is now which particle pairs and subsequent reactions are dominating this MFE. The possible mechanisms are currently divided into three categories: reactions of polarons with the same charge into bipolarons [15] , reactions of polarons with opposite charge into excitons [16] and reactions of triplet excitons with polarons [17] or with other triplet excitons [24] . We will refer to those mechanisms as bipolaron, electron–hole (e–h), triplet–polaron and triplet–triplet mechanism, respectively. Most experimental studies have focused on trying to isolate a certain mechanism, for example, by creating a device where only one type of polaron is present; however, a magnetoresistive response was always observed and no mechanism could be excluded. So far the largest effects have been observed in organic light-emitting materials and devices, where all particle reactions can potentially occur. To proactively unravel the underlying mechanism, an exquisite control of the spin-carrying particle interactions and subsequent magnetic field-dependent reactions is required. In this article, we propose a polymer-fullerene blend as most suitable candidate. Introducing fullerene to the polymer system enables a detailed control of the particle and spin interactions and provides a novel method to investigate the different mechanisms. At low concentration, the fullerene effectively quenches excitons into weakly bound, spatially separated charge-transfer (CT) states (CTSs), thereby reducing the exciton densities [25] , [26] . At higher concentration, phase separation additionally leads to separate electron and hole current pathways through the device [25] , [27] , [28] . Following earlier suggestions by Wang et al. [8] on MFEs in polymer-fullerene blends, we succeeded in fully correlating pronounced changes in the MFEs to the complementary (spin) physics in the different concentration regimes. Using detailed experimental analysis, explicit microscopic and numerical device simulations, we thus unravel the dominant underlying mechanisms of OMAR. In contrast to earlier work, our analysis allows us to quantitatively explain the observed linewidths and sign changes. Relevant OMAR mechanisms and their fingerprints A unified picture of the relevant particles and their (spin dependent) reactions is shown in Fig. 1 . The left panel shows possible polaron pairs in an organic semiconductor as a function of energy. Free charges can form precursor pairs in a singlet or triplet configuration. From this pair state, the precursor pair can either recombine into a singlet or triplet exciton (in the case of an e–h pair), a singlet bipolaron (in the case of a bipolaron pair) or dissociate back into free carriers again. Within the precursor pairs, the separation between the two carriers is such that exchange interactions are still negligible, enabling hf-induced mixing of the singlet and triplet precursor pairs [29] . An external magnetic field suppresses this mixing and thereby changes the transition to the singlet and triplet exciton or bipolaron state. Such a MFE governed by the hf strength, typically on the order of milliteslas, is referred to as a low field effect (LFE). Recently, it has been shown that the LFE can be accompanied by a distinct MFE at ultra-small field effect (USFE, ≤mT) scales [12] , [20] . 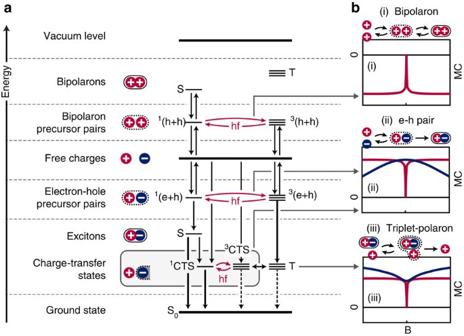Figure 1: Unified picture of relevant particles and their spin-dependent reactions. (a) Possible polaron pairs in an organic semiconductor as a function of energy. Free charges can form precursor pairs in a singlet (S)1( ) or triplet (T)3( ) configuration. From this pair state, the precursor pair can either recombine into a S or T exciton (in the case of an e–h pair), a S bipolaron (in the case of a bipolaron pair) or dissociate back into free carriers again. Because of hyperfine fields (hf) the S and T precursor pairs can mix and an external magnetic field can suppress this mixing. The magnetic field-dependent transitions between the pair states are indicated with curved arrows. The energy levels and possible mixing mechanisms of a CTS are also included in the diagram (shaded area). Electrons and holes are interchangeable in this diagram. (b) The characteristic low (red) and high (blue) field lineshapes of the (i) bipolaron, (ii) e–h and (iii) triplet–polaron mechanism, all according to explicit calculations using a density matrix formalism. Figure 1: Unified picture of relevant particles and their spin-dependent reactions. ( a ) Possible polaron pairs in an organic semiconductor as a function of energy. Free charges can form precursor pairs in a singlet (S) 1 ( ) or triplet (T) 3 ( ) configuration. From this pair state, the precursor pair can either recombine into a S or T exciton (in the case of an e–h pair), a S bipolaron (in the case of a bipolaron pair) or dissociate back into free carriers again. Because of hyperfine fields (hf) the S and T precursor pairs can mix and an external magnetic field can suppress this mixing. The magnetic field-dependent transitions between the pair states are indicated with curved arrows. The energy levels and possible mixing mechanisms of a CTS are also included in the diagram (shaded area). Electrons and holes are interchangeable in this diagram. ( b ) The characteristic low (red) and high (blue) field lineshapes of the (i) bipolaron, (ii) e–h and (iii) triplet–polaron mechanism, all according to explicit calculations using a density matrix formalism. Full size image The magnetic field-controlled transitions between singlet and triplet precursor pair states can have profound LFEs on the current through the organic semiconductor. First, within the bipolaron mechanism [15] , an external magnetic field will decrease the current by spin-blocking, an effect well known from low-temperature transport studies on double-quantum dot systems [30] . The bipolaron model treats the scenario where a charge carrier is quasi-stationary trapped at an energetically relatively low-lying state. A nearby free carrier, which contributes to the current, has to pass this site by—at least as a temporary intermediate state—forming a doubly occupied site, that is, a bipolaron. It should be noted that because of the large exchange within the bipolaron state, its formation is spin dependent. Therefore, it is well possible for a pair of polarons in a singlet configuration but very unlikely for the triplet, as depicted in Fig. 1a . Then, if the two carriers in the precursor pair are in a triplet configuration, the current is effectively blocked. At low magnetic fields, the spin-blocking is lifted due to the hfs efficiently mixing the precursor spin states, as indicated by the curved arrows in Fig. 1a . At high fields, blocking is regained, because random hfs are overruled, and spin character becomes well preserved. Thus, the bipolaron mechanism gives rise to a magnetic field dependence of the charge-carrier mobility μ and leads, in this case, to a negative magnetoconductance (MC). Next, within the e–h pair model as proposed by Prigodin et al. [16] , the crucial reaction is between weakly, Coulombically bound, e–h precursor pairs as shown in Fig. 1a . These pairs form statistically with a 1 (e+h): 3 (e+h) ratio of 1:3. They can dissociate to form free polarons, but can also react to form an exciton from where they finally can recombine to the ground state. If at least one of the two reactions is spin selective, the magnetic field will control the charge balance in the device, and thereby the current. Prigodin et al. [16] derived a magnetic field-dependent recombination rate, which was then linked to a so-called recombination mobility μ r . The authors assumed a different recombination rate for singlets and triplets. So, with less mixing due to a magnetic field, there is less recombination. In the space charge-limited (SCL) regime, this reduction leads to more current because of compensation of positive and negative space charge and thus gives rise to a positive MC [16] . In passing, we note that generally the e–h pair mechanism is unlikely to produce large MFEs, because it requires a competition between recombination and dissociation of precursor e–h pairs—that is, e–h pairs that in a single step can form an exciton. Usually, this is highly unlikely, because once the electron and hole have approached each other that close, they are well within the Coulomb radius, making dissociation a very unlikely event. However, in organic photovoltaic cells, the e–h pairs are in the form of CTSs, where dissociation does become relatively large [26] and, as we show, the e–h mechanism can result in significant MFEs. Lastly, we will discuss the triplet–polaron mechanism as first proposed by Desai et al. [17] In this model, triplet excitons can react with polarons by scattering events, which effectively reduce the mobility of the free charges and thereby decrease the current through the device. As triplet excitons in general have a much longer lifetime than singlet excitons, their concentration can become large enough so that these reactions become significant. By applying a magnetic field, less triplet excitons are formed, and thereby the current is increased, thus giving rise to a positive MC. We emphasize that even though the current is now influenced by the reaction of triplets with polarons, the LFE arises from the magnetic field-dependent formation of these triplet excitons. Therefore, the hyperfine-induced spin mixing of e–h precursor pairs, as indicated in Fig. 1a , is a crucial ingredient of the triplet–polaron mechanism. In addition to the LFEs, so-called high field effects (HFEs) occur at field scales much larger than the local hfs. Within the triplet–polaron model, spin mixing occurs between doublets (D) and quadruplets (Q) of triplet exciton–polaron pairs. Because of the zero-field splitting (ZFS, typically 80 mT (ref. 31 )) of the triplet exciton, the hf-induced spin mixing now manifests itself as a HFE at a broader linewidth. Using the same arguments as for the LFE, this HFE gives rise to a positive MC. The mutual annihilation of triplets also gives rise to a HFE with a linewidth determined by the ZFS [21] . However, because the triplet–triplet mechanism creates free charges, and an increasing magnetic field effectively reduces the amount of available triplets, this leads to a negative MC. A distinctly different HFE displays in the e–h mechanism. The opposite polarons in the e–h pair will generally have a (slightly) different g -factor, leading to dephasing of the precession electron and hole spins [29] . As a consequence, additional spin mixing occurs at large fields (typically 1 T), referred to as Δ g -mechanism. The associated HFE on the current will necessarily have a sign opposite to the corresponding LFE, which is based on the suppression of spin mixing. All the above-mentioned LFE and HFE mechanisms have been explicitly calculated using a density matrix formalism (also see Schellekens et al. [21] ), and the characteristic resulting MFE lineshapes are depicted in the right panel of Fig. 1b . For more details on these calculations, we refer to the Supplementary Note 1 . In passing, we note that other models—based on spin mixing by hfs—have been proposed in the literature. These models are mostly different implementations of one of the mechanisms as discussed before. For example, Harmon and Flatté [22] recently proposed a model that is a percolation implementation of the spin-blocking—or bipolaron—mechanism, whereas Hu and Wu [7] combined e–h pair mixing with triplet–polaron interactions and included dissociation processes. Besides hfs, other mixing mechanisms such as spin–orbit coupling have been proposed to explain OMAR [32] , [33] . However, for the organic materials that consist of low-molecular-weight organic semiconductors, as used in this work, this process is of minor relevance. Finally, completely different mechanisms have been introduced in the literature such as Lorentz-force deflection, hopping magnetoresistance or effects like weak localization and wave function shrinking [34] , [35] . However, most of them seemed not viable candidates to explain the effect or not needed to fully explain experimentally observed trends. Summarizing, the three mechanisms display clear fingerprints, with distinguishable characteristics such as sign and field scale of the LFE and HFE. These characteristics, which have been calculated and are schematically shown in Fig. 1b , will prove invaluable in identifying the relevant mechanisms. MFEs in polymer-fullerene blends In this study, we used a variety of blends, but most focus will be on blends of poly(2-methoxy-5-(3,7-dimethyloctyloxy)-1,4-phenylenevinylene) (MDMO-PPV):[6,6]-phenyl-C 61 -butyric acid methyl ester (PCBM), where PPV acts as hole-conducting polymer and electron donor, whereas PCBM acts as electron acceptor. This blend is a well-known and extensively studied organic photovoltaic system [25] , [26] , [27] , [28] , [36] , [37] , [38] , [39] , [40] , [41] , [42] , [43] . We will exploit the thorough understanding of the charge transport and morphology of this model system as a basis of our identification. We have systematically investigated the MFE on the current (MC) as a function of the applied magnetic field B and the bias voltage V for a broad range of PCBM concentrations x ; for the complete data set, we refer to Supplementary Fig. S2 in the Supplementary Information . We observed an extremely rich behaviour of the MFE with very pronounced changes in both the amplitudes and line widths. Typical results for three different concentrations x are shown in Fig. 2 . At low PCBM concentrations (0–10 wt.%, Fig. 2a ), we observe a positive LFE, which is accompanied by a positive HFE with a width on the order of 100 mT. The corresponding USFE is shown in Fig. 2b . In sharp contrast, at intermediate concentrations (30–60 wt.%, Fig. 2c ), a positive LFE and an opposite (negative) HFE at much larger field scale (~1 T) are observed. When increasing the PCBM content over 70%, all MC curves only show a negative LFE and almost no HFE. Based on these fingerprints, we raise the hypothesis that the triplet–polaron, e–h and bipolaron mechanism, respectively, are the dominant underlying mechanisms. This conjecture will be put on more solid ground using quantitative arguments in the remainder of this article. 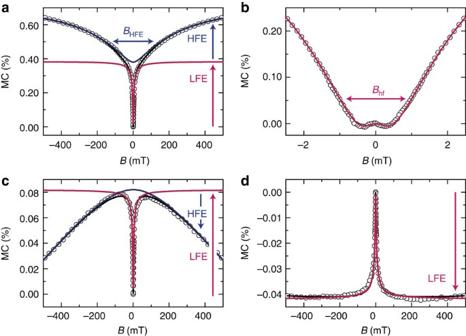Figure 2: MFE on the current as a function of the applied magnetic field. (a) The MFE for a 1 wt.% MDMO-PPV1−x−PCBMxblend at 3.0 V. The solid line is a fit using the empirical lineshape (see Methods section), where the LFE and HFE contributions are separately depicted. The magnitude of LFE and HFE and their corresponding line widthsBhfandBHFEare also shown. (b) At low magnetic fields, on the order of a millitesla, an USFE appears which is also correctly described by the fit. (c) The MFE for a 50% blend at 1.1 V. Here the LFE and HFE have a different sign, and the line width of the HFE is much broader. (d) The MFE for a 80% blend at 1.1 V, showing a negative LFE and almost no HFE. Figure 2: MFE on the current as a function of the applied magnetic field. ( a ) The MFE for a 1 wt.% MDMO-PPV 1−x −PCBM x blend at 3.0 V. The solid line is a fit using the empirical lineshape (see Methods section), where the LFE and HFE contributions are separately depicted. The magnitude of LFE and HFE and their corresponding line widths B hf and B HFE are also shown. ( b ) At low magnetic fields, on the order of a millitesla, an USFE appears which is also correctly described by the fit. ( c ) The MFE for a 50% blend at 1.1 V. Here the LFE and HFE have a different sign, and the line width of the HFE is much broader. ( d ) The MFE for a 80% blend at 1.1 V, showing a negative LFE and almost no HFE. Full size image Analysing the MFE We performed a detailed analysis of the experimental results by fitting the MC ( B ) data at all x and V , with a superposition of a LFE (including USFE) and a HFE (see Methods and Wagemans et al. [44] ). Thus, for each measurement, we get an amplitude of the LFE and HFE, but also the intrinsic hf scale ( B hf ), as well as the half-width at quarter-height of the HFE ( B HFE ). The extracted parameters are shown in Fig. 3 . 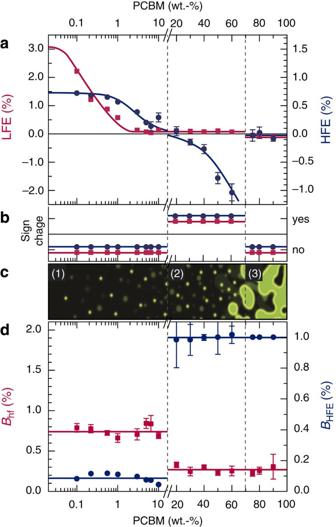Figure 3: Global trends of the MFEs in the current. (a) The top figure shows the maximum value of the magnitude of the MC for the low (LFE, left axis, red squares) and high MFE (HFE, right axis, blue circles) as a function of PCBM content at voltages higher than the built-in voltageVbi. The lines provide a guide to the eye. (b) This panel shows if there is a sign change in the MFE as a function of voltage. (c) An illustration of the morphology of the organic layer with the three distinct regions indicated. (d) The bottom figure shows the width of the two MFEs (BhfandBHFE). The error bars represent the uncertainty in the fitting values. Figure 3a presents the maximum observed magnitude of the LFE and HFE in each specific blend, whereas the line widths are shown in Fig. 3d . In both figures, we observe very pronounced trends, which can be correlated with different morphology regimes of the polymer–PCBM blend [27] , schematically represented in Fig. 3c . Figure 3: Global trends of the MFEs in the current. ( a ) The top figure shows the maximum value of the magnitude of the MC for the low (LFE, left axis, red squares) and high MFE (HFE, right axis, blue circles) as a function of PCBM content at voltages higher than the built-in voltage V bi . The lines provide a guide to the eye. ( b ) This panel shows if there is a sign change in the MFE as a function of voltage. ( c ) An illustration of the morphology of the organic layer with the three distinct regions indicated. ( d ) The bottom figure shows the width of the two MFEs ( B hf and B HFE ). The error bars represent the uncertainty in the fitting values. Full size image Initially, at small x , regime (1) in Fig. 3c , PCBM will form scattered (clusters of) molecules in the PPV matrix, providing efficient quenching sites for excitons and introducing CTSs with holes residing on the polymer and electrons on the PCBM. Beyond x =20%, regime (2), a perculative network for electron conduction along PCBM molecules forms. Importantly, the electrons remain in intimate contact with holes in the PPV matrix. When increasing x beyond 70%, regime (3), phase separation occurs, creating separate regions dominated by single-carrier electron and hole currents. The exact concentration at which this happens for our blends is known from the literature [27] , but has also been verified by means of atomic force microscopy (see Supplementary Fig. S3 ). Very interestingly, pronounced changes in Fig. 3a,d , such as sign changes and abrupt changes in linewidths, exactly correlate with boundaries between the three morphology regimes. We start our discussion with regime (1). In the pristine polymer, triplet exciton densities can be very high because of the long triplet lifetime, making the triplet–polaron mechanism a likely candidate. The positive sign of the LFE and the width of the HFE (~80 mT), a typical value for the ZFS [31] , is consistent with this interpretation. Very remarkably, we observe that the magnitude of both the LFE and HFE are quenched by adding just a few wt.% PCBM, consistent with PCBM acting as an efficient quencher of excitons. Note that the LFE responds more sensitively to adding PCBM, which can be assigned to the relative alignment of CT and triplet exciton energy as is discussed in detail in the Supplementary Note 2 . Next, we will discuss regime (2). In these blends, PCBM is still homogeneously distributed throughout the PPV but forms percolative current paths for electrons [27] . Excitons are effectively quenched and transferred into CT pairs, which in our blend are known to be energetically aligned with the triplet excitons on the PPV ( Fig. 1a ) (refs 40 , 41 ). This would provide an ideal scenario for an electron (on PCBM)–hole (on PPV) pair-mediated mechanism, for which it is necessary that there is a finite chance for e–h pair formation as well as dissociation. Indeed, the observation of a sign change to a negative HFE, as well as an abrupt change to a large field scale due to a Δ g -mechanism when entering regime (2), corroborates this assignment. The field scale of approximately 1 T agrees with the field scale that we calculated based on experimental values of g e =1.9995 and g h =2.0028 (refs 36 , 37 , 38 ). Even more excitingly, a sudden and significant reduction of B hf , as extracted from the LFE, can be witnessed. This is naturally explained by the very small hf coupling that electrons experience on the fullerene cages due to the vanishing nuclear magnetic moment of 12 C. Finally, in regime (3) the blends are separated into two phases. The electrons are primarily transported through a PCBM phase, and the holes are transported through a mixed phase of PPV and PCBM [27] , [28] . With separate current paths for electrons and holes, locally the device will perform as a single-carrier device. Thus, the bipolaron mechanism, the only mechanism not relying on charge carriers with opposite charges, is expected to become dominant over the e–h pair mechanism in phase-separated blends. Indeed, we observe the LFE changing to a negative value and we observe a quenching of the HFE caused by the Δ g -mechanism. After this satisfactory identification of the dominant mechanisms in all three regimes, we show that we can also quantitatively describe the voltage dependence and that specific features herein are in full agreement with our assignment. As such, this provides an alternative route towards unravelling underlying mechanisms. To do so, we performed finite element drift-diffusion simulations [19] , [31] , [38] , [41] for realistic parameters (please refer to the Supplementary Note 3 for more details). Here we will briefly discuss the MC( V ) in all three regimes, starting with regime (2). In Fig. 3b it is displayed whether at a certain x , a sign change in MC( V ) is observed in LFE and HFE. Apparently, regime (2), dominated by the e–h mechanism, is a special regime, where experiments on both the LFE and HFE show a sign change. The experimental LFE( V ) and current density, J ( V ), are plotted in Fig. 4b,d , respectively. Therefore, it gets clear that the sign change in the LFE occurs around the built-in voltage V bi , where the current undergoes a transition from the (exponential) diode-like diffusion regime to the (power law) SCL drift regime [25] . 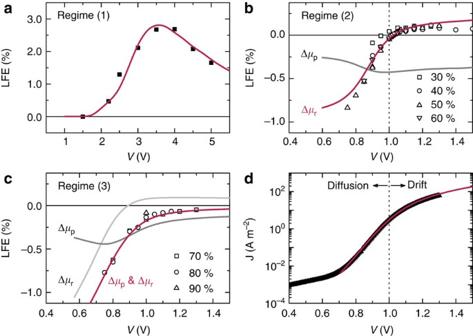Figure 4: Experimental and simulated voltage dependencies. Experimental (symbols) and simulated (solid line) LFE as a function of voltage for (a) pristine devices, (b) homogenous mixed blends in regime (2) and (c) the phase-separated blends in regime (3). (d) Experimental (symbols) and simulated (solid line) current density as a function of voltage for a 50 wt.% blend showing a transition from a diffusion to drift dominated regime around the built-in voltage. Figure 4: Experimental and simulated voltage dependencies. Experimental (symbols) and simulated (solid line) LFE as a function of voltage for ( a ) pristine devices, ( b ) homogenous mixed blends in regime (2) and ( c ) the phase-separated blends in regime (3). ( d ) Experimental (symbols) and simulated (solid line) current density as a function of voltage for a 50 wt.% blend showing a transition from a diffusion to drift dominated regime around the built-in voltage. Full size image We can provide an intuitive explanation for the sign change. In the drift regime, enhancing recombination by applying a magnetic field reduces space charge compensation of the electron and hole currents and hence reduces the current of bipolar SCL devices, whereas in the diffusion regime carriers recombining in the ‘depletion zone’ of the diode enhance the current. To quantify this prediction, we performed simulations for devices consisting of homogeneous blends of the polymer and fullerene. The calculated current density, as shown in Fig. 4d , matches the experimental result using realistic parameters [39] , [42] . We also explicitly calculated the MFEs by assuming a change in the recombination mobility Δ μ r , or hole mobility Δ μ p . The results of these simulations are depicted in Fig. 4b . Here, it is clear that the sign change around V bi is readily reproduced in the case of a change in recombination mobility, strengthening our conclusion that the e–h mechanism is dominant in this regime. In regime (3), a rather similar dependence of the LFE is observed ( Fig. 4c ), however, without the characteristic sign change. Explicit simulations show that this can be traced back to the superposition of an almost constant and negative MC( V ) due to the bipolaron mechanism (realized by a change in carrier mobility Δ μ p ) and a finite contribution from the e–h mechanism (change in recombination mobility Δ μ r ). The latter contribution is most probably related to the interaction of electrons and holes at the interface between the two phases in the blend, an effect which our device simulations take into account [39] , [42] . Also regime (1) shows a very characteristic MC( V ) dependence ( Fig. 4a ), vanishing below the built-in voltage and peaking somewhat above. A full description of those dependencies goes beyond the scope of our present article, but more information on the calculation is provided in the Supplementary Note 3 . Here we will briefly discuss these recent advances, where trap states have an important role. We found that we can numerically simulate the MC( V ) trend with a trapped triplet–polaron mechanism, as is shown in Fig. 4a . This mechanism involves the spin-dependent formation of triplet excitons at trap sites and their subsequent reaction with free polarons. A magnetic field will reduce the number of triplets and thereby enhance the number of free polarons. The initial increase of the MC( V ) then simply stems from the increase of triplet density with voltage, whereas the eventual decrease arises from the fact that there is only a limited number of traps available in a device. Finally, as an outlook, we conjecture that by choosing the right materials to alter the alignment of triplet excitons and CTSs or intentionally introducing specific trap sites [14] , [45] , huge effects on the reaction pathways and the resulting OMAR can be achieved. As an example of the former, we are currently investigating polymer-fullerene blends using different material combinations. A result for two different polymers is shown in Fig. 5 , where we have added 5 wt.% PCBM to the regular MDMO-PPV ( Fig. 5a,b ) and a phenyl-substituted poly(1,4-phenylenevinylene) polymer called SY-PPV ( Fig. 5c,d ). We observe a distinctly different lineshape at low magnetic fields, revealing an additional negative LFE. 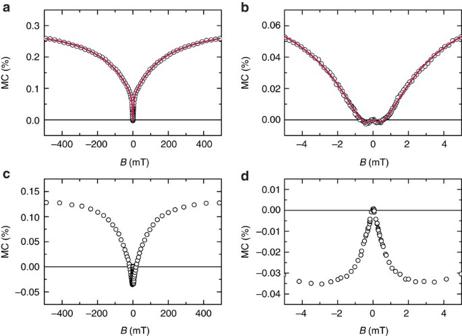Figure 5: MFE for two different polymers-fullerene blends. (a,b) The top panels show the result for a 5 wt.% MDMO-PPV:PCBM blend, whereas (c,d) the bottom panels show the result for a 5 wt.% SY-PPV:PCBM blend. The right panels present a zoom around zero applied field, showing a distinct additional negative contribution appearing in the SY-PPV blends. This contribution is not observed in the MDMO-PPV blends. Figure 5: MFE for two different polymers-fullerene blends. ( a , b ) The top panels show the result for a 5 wt.% MDMO-PPV:PCBM blend, whereas ( c , d ) the bottom panels show the result for a 5 wt.% SY-PPV:PCBM blend. The right panels present a zoom around zero applied field, showing a distinct additional negative contribution appearing in the SY-PPV blends. This contribution is not observed in the MDMO-PPV blends. Full size image We can explain this contribution by a small shift in the energetic alignment of the CTS with respect to the triplet exciton as illustrated in Fig. 6 . In a large applied magnetic field ( Fig. 6a ), additional triplet excitons are created by process (3). Without an external field, spin mixing of the CTS, indicated by process (2) in Fig. 6b , leads to a reduction of process (3). In other words, applying a magnetic field leads to more triplet excitons and thereby less current due to scattering of triplet excitons with charges, and consequently thus a negative MC. The insights obtained in our present work seem invaluable in understanding these novel MFEs. 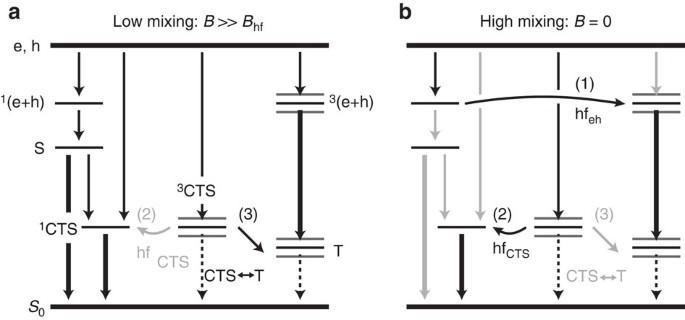Figure 6: Fastest relevant recombination routes in a different polymer-fullerene blend. Here the CTS is higher in energy than the triplet state in the polymer: (a) in a large external magnetic field and (b) in the absence of an external magnetic field. Processes (1) and (3) lead to an increase in triplet (T) in the absence of an external field, while process (2) decreases T. Figure 6: Fastest relevant recombination routes in a different polymer-fullerene blend. Here the CTS is higher in energy than the triplet state in the polymer: ( a ) in a large external magnetic field and ( b ) in the absence of an external magnetic field. Processes (1) and (3) lead to an increase in triplet (T) in the absence of an external field, while process (2) decreases T. Full size image Concluding, in this article we presented a proof of concept study, unravelling the role of the relevant particle pairs and their reactions for OMAR. Furthermore, we explained how striking differences in the MFE lineshapes are correlated with the underlying microscopic mechanisms and have shown the important role of device physics. Our findings open up unprecedented means to bring OMAR research from a phase of passively observing MFEs in the current, to really engineering device characteristics by tailoring the molecular system. Samples In this work, we studied the MFEs on the current for devices consisting of a blend of MDMO-PPV and PCBM. The MDMO-PPV was purchased from American Dye Source Inc. and the PCBM (>99% pure) from Solenne B.V. The devices were prepared on glass substrates with patterned indium tin oxide (ITO) anodes. After careful cleaning, followed by a ultraviolet-ozone treatment, a thin layer of poly(3,4-ethylenedioxythipophene):poly(styrenesulfonate) (PEDOT:PSS) was applied by spin coating. The MDMO-PPV and PCBM were both dissolved in orthodichlorobenzene, with a concentration of 10 and 20 mg ml −1 , respectively, and stirred on a hot plate at 50 °C for at least 2 h after appropriate blending. The blends were spin coated at 1,200 r.p.m. for 60 s. Subsequently, the samples were transferred to a nitrogen-filled glove box where the cathode, consisting of LiF and Al, was evaporated in a high-vacuum system (~10 −7 mbar). From this point on, the samples always remain in a dry nitrogen environment. The total junction stack thus consisted of ITO/PEDOT:PSS (60 nm)/[PPV 1− x −PCBM x ] (~80 nm)/LiF (1 nm)/Al (100 nm), with the PCBM concentration x in wt.%. Measurements MFE measurements were performed in a cryostat that is attached to a glove box with a nitrogen environment ([O 2 ] <0.3 p.p.m., [H 2 O] <0.3 p.p.m.). The cryostat is placed between the poles of an electromagnet. The measurements described in this article were performed at room temperature. The devices were driven at a constant voltage V using a Keithley 2400 Series SourceMeter. We measured the current I through the device while sweeping the magnetic field B. From this measurement, the MC was calculated with MC ( B )=( I ( B )− I (0))/ I (0). Empirical lineshapes We have analysed our experimental results using the following fitting function: . The function is explained in full detail by Wagemans et al. [44] and is used to correctly describe the LFE including the USFE as shown in Fig. 2b . This empirical function allows us to separately extract the role of the hf ( B hf ) and the additional broadening ( B m ) induced by the microscopic mechanisms involved. The USFE is incorporated by the parameter r that describes the limit in which hopping of carriers is no longer slow compared with spin precession in the hfs. The HFE is fitted with a so-called non-Lorentzian lineshape. In the fitting procedure, for each specific blend x , the line widths ( B hf , B m and B HFE ) were shared fit parameters, whereas the magnitudes (LFE and HFE) and the hopping ratio ( r ) were free fit parameters. In this study, we investigated the amplitudes and line widths. The discussion of the other fitting parameters, although extracted and analysed, is beyond the scope of the present work. How to cite this article: Janssen, P. et al. Tuning organic magnetoresistance in polymer-fullerene blends by controlling spin reaction pathways. Nat. Commun. 4:2286 doi: 10.1038/ncomms3286 (2013).